High-strength carbon nanotube fibre-like ribbon with high ductility and high electrical conductivity Macroscopic fibres made up of carbon nanotubes exhibit properties far below theoretical predictions and even much lower than those for conventional carbon fibres. Here we report improvements of mechanical and electrical properties by more than one order of magnitude by pressurized rolling. Our carbon nanotubes self-assemble to a hollow macroscopic cylinder in a tube reactor operated at high temperature and then condense in water or ethanol to form a fibre, which is continually spooled in an open-air environment. This initial fibre is densified by rolling under pressure, leading to a combination of high tensile strength (3.76–5.53 GPa), high tensile ductility (8–13%) and high electrical conductivity ((1.82–2.24) × 10 4 S cm −1 ). Our study therefore demonstrates strategies for future performance maximization and the very considerable potential of carbon nanotube assemblies for high-end uses. Current development of fibrous materials has focused on increased functionality and performance by means of concurrent maximization of both mechanical and physical properties required for many applications. To this end, carbon fibre has achieved partial success as some CFs have a tensile strength σ b reaching 6 GPa, and others an electrical conductivity κ approaching 1.0 × 10 4 S cm −1 (see ref. 1 ). But deficiencies of their own virtues do exist, mainly including: (1) a low tensile elongation to break ( δ , ~1–2%) and very low κ for high-strength CFs and (2) low σ b and even nil δ for high-conductivity CFs. Such deficiencies have excluded CFs to be used in the areas where plasticity and conductivity are particularly demanded as safety and performance design factors. Carbon nanotubes (CNT) combine the best properties of polymers, CFs and metals, resulting from their strong carbon–carbon covalent bonds and unique atomistic structures. For example, the σ b and δ for individual CNTs are in the ranges of 11 GPa–63 GPa and 10%–30%, respectively [2] , [3] . The κ is as high as 10 6 S cm −1 for single-walled CNTs [4] and 3 × 10 4 S cm −1 for multiwalled ones [5] . In order to fully utilize these excellent axial properties at a macroscopic level, CNTs must be assembled to form macroscopic fibres. A key issue in the assembling is to align the CNTs along the fibre axis and pack them as densely as possible. But, this remains as a daunting challenge to fibre fabrication and processing for materials scientists and engineers. To date, there are three methods for producing CNT fibres continuously (see recent reviews [6] , [7] ). The first method is spinning from CNT solutions [8] , [9] , [10] . Post-treatments, such as hot-drawing, enhanced nanotube alignment and hence mechanical performance [11] , [12] . Recent spinning of ~5-μm long CNTs improved Young’s modulus E to 120 GPa, σ b to 1.0 GPa, κ to 2.9 × 10 4 S cm −1 , but with δ as low as 1.4% (ref. 13 ). The second method is spinning from vertically aligned CNT arrays [14] , [15] , [16] . Introducing twisting [15] , tension [17] , [18] or liquid shrinking during drawing [16] , [19] aligns and/or compacts the CNTs. Post treatment of twisting led to 1.9 GPa for σ b , 7% for δ and 4.1 × 10 2 S cm −1 for κ [20] , but that of twistless rubbing resulted in a porous structure in the fibre [21] . The third method is spinning from a CNT aerogel formed in a high-temperature reactor [22] , [23] , [24] . Increasing the spinning rate and densifying the fibre in acetone vapour enhanced CNT alignment and fibre density, respectively. The reported best σ b is up to 1.25 GPa, δ to 18% and κ to 5 × 10 3 S cm −1 (ref. 25 ), although higher σ b was recorded from testing at 1 and 2 mm gauge lengths (GLs) [24] , [26] . Although significant progress has been made, the mechanical and physical properties of CNT fibres measured to date are still far below those for individual CNTs and even much lower than those for commercial CFs. Here, we report a general strategy for performance maximization. It is shown that the initial CNT fibre spun from a hollow macroscopic cylinder can be densified by mechanical rolling under pressure, and such densification can lead to improvements of mechanical and electrical properties by more than one order of magnitude. The achieved combination of a high strength (4.34 GPa), a high ductility (10%) and a high electrical conductivity (2 × 10 4 S cm −1 ) is superior to those for any other fibres and films currently available, and thus suggests the potential of CNT assemblies for wide applications. Continuous spinning process A schematic and results of our spinning process are shown in Fig. 1 . The reaction solution was injected into the reactor for pyrolysis. CNTs formed in the high-temperature zone and integrated into a film in the low-temperature region. Modulating the composition and feeding rate of the precursor solution and the flow rate of the carrier gas of nitrogen is of primary importance to form a cylindrical film based on the inner wall of the tube reactor and extrude this film out continuously ( Fig. 1b ). See Supplementary Movies 1 and 2 for the continuous flow of a CNT cylinder from the reactor. 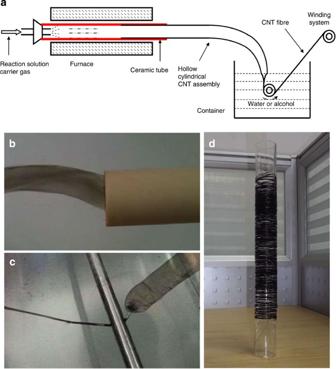Figure 1: Experimental set-up and results. (a) Reaction solution is sprayed into a tube reactor and pyrolysized to form carbon nanotubes (CNTs). (b) CNTs self-assemble to a hollow cylinder, which is blown out from the reactor. (c) The cylindrical assembly is condensed in water or alcohol, and the resultant fibre is pulled out. (d) The fibre is winded and collected on a glass tube. Figure 1: Experimental set-up and results. ( a ) Reaction solution is sprayed into a tube reactor and pyrolysized to form carbon nanotubes (CNTs). ( b ) CNTs self-assemble to a hollow cylinder, which is blown out from the reactor. ( c ) The cylindrical assembly is condensed in water or alcohol, and the resultant fibre is pulled out. ( d ) The fibre is winded and collected on a glass tube. Full size image We operated the condensation process in an open-air environment. The CNT cylinder could be condensed by spraying acetone on it, and the resultant fibre winded up as done before [24] . But, we found that, in order to achieve good condensation, the spraying had to be sufficiently heavy. The heavy spraying of flammable acetone in open air not only induced safety issue but also disturbed the continuous flow of the cylinder from the reactor. Instead, we introduced the cylinder into a water or ethanol pool for condensation, captured the fibre underneath a rotating stainless steel rod ( Fig. 1c ). See Supplementary Movies 3 and 4 for the continuous condensation of the cylinder to a fibre. The fibre could be winded on the rotating rod in the pool and unwinded later on ( Supplementary Fig. 1 ) or pulled out and winded outside on a glass tube ( Fig. 1d ) or any other mandrel driven by a speed-controllable motor. As the hollow cylinder was full of gases, a small force was needed to introduce it into the pool and pull the fibre out for winding. Such a force was certainly beneficial to stretch the fibre and align the inside CNTs. The winding rate that was in match to the running rate of the cylinder, was typically ~10 m min −1 . Structure and property of initial fibre The cylinder consisted primarily of CNTs, which are partially aligned along the cylinder axis ( Fig. 2a ). Efforts were ever made to track the length of the CNTs under scanning electron microscopy (SEM), but no clear results were obtained as ends were seldom seen, presumably because of their long length and mutual entanglement. The content of Fe particles was generally low ( Fig. 2b ). Quantitative estimation by thermo-gravimetric analysis (TGA) revealed its variation in the range from 7 to 15 wt.%, depending upon the amount of ferrocene added. The constituent CNTs were mainly double walled with some being other thin walled with diameters in the range of 2–7 nm ( Fig. 2c ). Raman spectroscopy showed a high ratio (3.74) of the intensity of the G peak (~1584, cm −1 ) to that of the D peak (~1325, cm −1 ; I G / I D ; Fig. 2d ), indicating a low density of sp 3 carbon defects in the nanotube sidewalls. 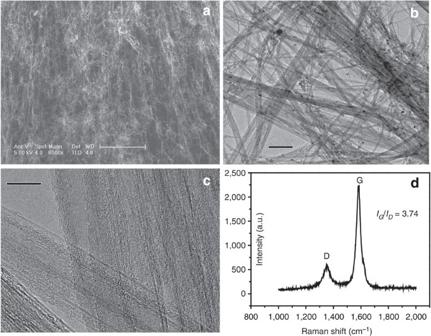Figure 2: CNT characterization. (a) SEM micrograph of the CNTs after the condensation of the hollow cylinder on a flat surface. (b) Transmission electron microscopy micrograph of the CNTs after ultrasonic separation from the cylinder. (c) High-resolution transmission electron microscopy micrograph of the thin-walled CNTs. (d) Raman spectrum of the CNT fibre. Scale bars, 10 μm (a), 0.2 μm (b) and 10 nm (c). Figure 2: CNT characterization. ( a ) SEM micrograph of the CNTs after the condensation of the hollow cylinder on a flat surface. ( b ) Transmission electron microscopy micrograph of the CNTs after ultrasonic separation from the cylinder. ( c ) High-resolution transmission electron microscopy micrograph of the thin-walled CNTs. ( d ) Raman spectrum of the CNT fibre. Scale bars, 10 μm ( a ), 0.2 μm ( b ) and 10 nm ( c ). Full size image The fibre pulled from the pool had a rectangular, rather than a circular cross section at a microscopic scale. This apparently resulted from the reshaping of the fibre underneath the steel rod under the action of the winding force. The dimension of the cross section (width × thickness) was dependent on the diameter of the reactor tube and the liquid used for condensation. When a Φ40 mm reactor was used, the water-condensed fibre showed a width of ~160 μm but a thickness in the range of 5–9 μm, an uneven surface and porous interior ( Fig. 3a,b ). In the ethanol-condensed case, the fibre had a cross section of a low aspect ratio (~45 × 20 μm) with an even surface ( Fig. 3c ) and also a porous interior ( Fig. 3d , Supplementary Fig. 2 ). The differences between these two fibres are related to the different extents of shrinking induced by water and ethanol. 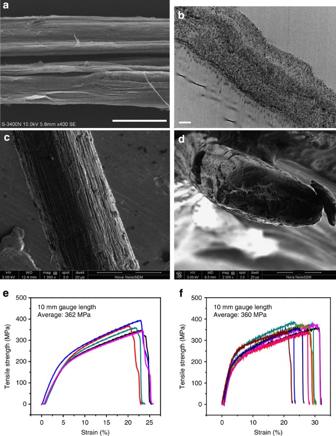Figure 3: Structure and mechanical property of initial fibre. (a) The surface and (b) cross section of water-condensed fibre. (c) The surface and (d) cross section of ethanol-condensed fibre. (e) Tensile stress versus strain curves of water-condensed fibre. (f) Tensile stress versus strain curves of ethanol-condensed fibre. The image inbis the cross section of the fibre embedded in epoxy and viewed in transmission electron microscopy. CNTs are seen as dark dots surrounded by epoxy as light grey regions. Due to epoxy impregnation, the pores were filled with the thickness slightly expanded. Scale bars, 100 μm (a), 2 μm (b), 40 μm (c) and 20 μm (d). Figure 3: Structure and mechanical property of initial fibre. ( a ) The surface and ( b ) cross section of water-condensed fibre. ( c ) The surface and ( d ) cross section of ethanol-condensed fibre. ( e ) Tensile stress versus strain curves of water-condensed fibre. ( f ) Tensile stress versus strain curves of ethanol-condensed fibre. The image in b is the cross section of the fibre embedded in epoxy and viewed in transmission electron microscopy. CNTs are seen as dark dots surrounded by epoxy as light grey regions. Due to epoxy impregnation, the pores were filled with the thickness slightly expanded. Scale bars, 100 μm ( a ), 2 μm ( b ), 40 μm ( c ) and 20 μm ( d ). Full size image Mechanical testing revealed a transition from an elastic response (linear stress versus strain) to plastic deformation (decreasing slope of stress versus strain) before failure, and an ultimate tensile strength of only 362 MPa and elongation of 20–30% ( Fig. 3e,f ). The water and ethanol-condensed fibres exhibited similar cross-sectional areas and ultimate loads, and thus similar ultimate stresses. The large fracture strain inherent with both fibres was evidently a result of CNT sliding over each other even in the presence of big pores ( Supplementary Fig. 3 ). Structures after rolling As the CNT packing in the fibre was loose after condensation in water or even alcohol, increasing packing density was critical for property improvement. To do this, we introduced pressurized rolling to the fibre, and repeated the rolling for up to five times ( Fig. 4a ). Insufficient rolling generated inhomogeneous surface morphologies, but excessive rolling resulted in damage to the fibre. We performed rolling on water-condensed fibres, but not on ethanol-condensed ones. Our preference was based on the considerations that (1) water is more environment friendly with no risk catching a fire than ethanol and (2) fibres had a much larger aspect ratio in cross section so that it was possible to orient the fibre on the roller and roll it always at its thickness direction. 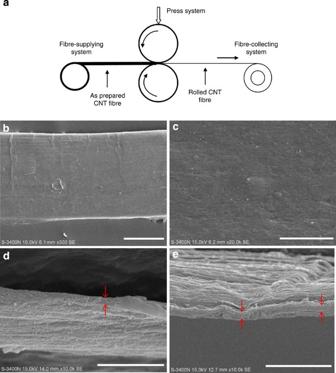Figure 4: Surface structure after pressurized rolling. (a) A schematic of the system for rolling carbon nanotube (CNT) fiber. (b,c) SEM images of the sample after rolling, showing a smooth surface morphology. (d) SEM image of the sample being tilted toward viewer. (e) SEM image of the sample being nearly horizontal with the front cross section slightly folded upward. Arrowed indandeare the sample thicknesses. Scale bars, 100 μm (b), 2 μm (c) and 5 μm (d,e). Figure 4: Surface structure after pressurized rolling. ( a ) A schematic of the system for rolling carbon nanotube (CNT) fiber. ( b , c ) SEM images of the sample after rolling, showing a smooth surface morphology. ( d ) SEM image of the sample being tilted toward viewer. ( e ) SEM image of the sample being nearly horizontal with the front cross section slightly folded upward. Arrowed in d and e are the sample thicknesses. Scale bars, 100 μm ( b ), 2 μm ( c ) and 5 μm ( d , e ). Full size image SEM examination showed that after rolling, the fibre surface appeared smooth and only few previous pores were visible even at high magnification ( Fig. 4b,c ). While the width of the fibre increased only slightly from 160 to ~220 μm ( Fig. 4b ), the thickness reduced significantly from 5–9 μm to 500 nm ( Fig. 4d,e ), giving rise to a reduction of the cross-sectional area by a factor of ~10. The thickness of 500 nm may represent the upper limit as smaller thicknesses were also observed from time to time. Considering its long length of hundreds of metres at macroscopic scale but large cross-sectional aspect ratio and very thin thickness at microscopic level, the CNT assembly after rolling may be better described as a fibre-like ribbon. It was difficult to accurately determine the density of the assembly because of its low weight and structural change along its length. Weighing the rolled assembly of tens of metres long on a submicro balance led to densities varying from 1.3 to 1.8 g cm −3 . The estimated density was larger than those for fibres spun from solutions (1.3 g cm −3 ) [13] and aerogels (0.9 g cm −3 ) [24] . It was even sometimes larger than the theoretical density of CNTs (1.5 g cm −3 ) [13] and approached that for pure CFs (1.8 g cm −3 ) [1] . The additional mass may be due to the presence of iron catalyst particles from synthesis process. On the basis of wide-angle X-ray diffraction results ( Supplementary Fig. 4 ), the measured degrees of CNT alignment were 80.6 % and 82.6% for the as-spun and rolled samples, respectively. These measurements indicate a high percentage of individual CNTs were aligned along the fibre axis, and rolling did not induce significant change in CNT alignment. Properties after rolling Tensile testing exhibited exciting results ( Fig. 5 ). After repeated rolling, the ultimate tensile load increased only slightly (up to 1.2 times). At 10 mm GL, the average E was 91 GPa, and the ultimate σ b reached 3.76–5.53 GPa with an average of 4.34 GPa, a factor of 12 higher than that for the unrolled counterpart. This drastic enhancement is evidently largely due to the reduction of the cross-sectional area with a minor contribution for load increase. In order to examine the uniformity of the fibre-like ribbon, we tested the samples also at 1, 5 and 20 mm GLs ( Fig. 5 ). While the tensile strength was about the same, the tensile elongation decreased from ~27% at 1 mm GL to ~10% at 5 and 10 GLs and to the lowest of ~5% at 20 mm GL. At the same GL of 10 mm, rolling induced reduction in tensile elongation from ~25 to ~10%. 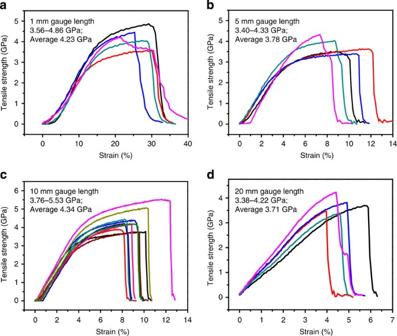Figure 5: Stress versus strain curves for rolled ribbons measured at different gauge lengths. (a) 1 mm, (b) 5 mm, (c) 10 mm, and (d) 20 mm. Figure 5: Stress versus strain curves for rolled ribbons measured at different gauge lengths. ( a ) 1 mm, ( b ) 5 mm, ( c ) 10 mm, and ( d ) 20 mm. Full size image In addition to the above mechanical properties, electrical conductivity was also measured for the same CNT assemblies. For the as-prepared sample, the conductivity varied slightly with the composition of the precursor solution (for example, water, ferrocene and thiophene additions) and experimental temperature. All measurements generated values around 1.27 × 10 3 S cm −1 . Rolling induced a significant increase in conductivity. For the ribbons with the mechanical properties described above, the conductivity was 1.82–2.27 × 10 4 S cm −1 , which is close to the theoretical value of 3 × 10 4 S cm −1 for multiwalled CNTs. The unique feature of the present approach is spinning the CNT assembly in open-air environment. Successfully avoiding previous uses of H 2 carrier gas and heavy alcohol spraying [22] , [23] , [24] are favourable for overcoming safety and environmental issues. Eliminating vacuum or sealed system is useful for processing the CNT cylinder in different ways. In addition, our fibre was spun from CNT cylinders. CNTs in these cylinders are more strongly integrated than those in aerogels and thus more suitable for continuous pulling and spinning even in the presence of turbulence. All these would add benefits for flexibility and easy scale-up. The main advance of the present study is the significant increase in packing density and thus mechanical and electrical properties by rolling. CNT fibres, especially those produced from CNT aerogels and arrays so far usually have low packing, and liquid shrinking and twisting are often used for densification, but the achieved properties are still unsatisfactory. Liquid shrinking cannot make uniform contraction at the radial direction of the fibre. Twisting, while bringing CNTs in closer contact with each other, introduces new voids and deviation of the axial load on CNTs from the external load applied on the fibre. So, the resultant twisting effect depends on the competition between its positive and negative contributions, which often leads to low net property improvement. We fully used the unique property of compressibility of CNTs to densify the CNT assembly. Both theoretical calculations [27] and experimental study [28] suggested that CNTs could bear substantial compression with their structures remaining intact. Thus, it is possible that during the present rolling, the pores and gaps between thin-walled CNTs could have gradually been eliminated as more and more rollings were imposed, generating an unprecedented packing in the assembly. As a result of the high packing, the present CNT assembly has an exceptional combination of high strength, high ductility and high conductivity. The main results for previous fibres made by the leading methods are listed in Supplementary Table 1 and illustrated in Fig. 6 . For neat fibres that are composed solely of CNTs, σ b varies over a very wide range. Inspection of Fig. 6a elucidates that previous neat fibres had σ b up to 1.9 GPa and δ to 9% (ref. 20 , 29 ) or lower σ b of 1.25 GPa but higher δ of 18% (ref. 25 ) although twisting was imposed for densification. Nevertheless, the present fibre has a much higher σ b of 3.76–5.53 GPa with a high δ of 8–13%. Moreover, the high σ b was measured at all GLs of 1, 5, 10 and 20 mm, indicating a homogeneous fibre and its extrinsic strength. Such an improvement evidently originates from the densification induced by repeated rolling. It remains as an eager expectation whether or not previous CNT fibres will also show a drastic improvement when similar rolling is applied. 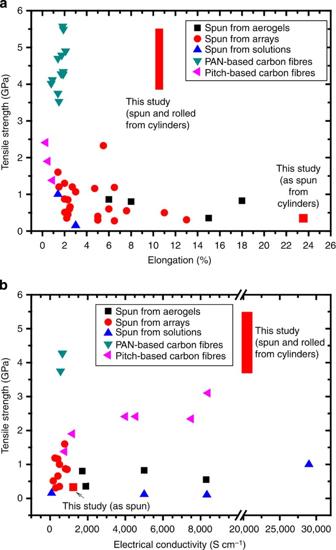Figure 6: Property comparisons between the present and previous carbon nanotube fibers. Data are based onSupplementary Table 1with the exclusion of composite and doped/coated fibers. Conventional carbon fibers based on pitch and polyacrylonitrile (PAN) are also included. (a) Mechanical property. (b) Electrical property. Figure 6: Property comparisons between the present and previous carbon nanotube fibers. Data are based on Supplementary Table 1 with the exclusion of composite and doped/coated fibers. Conventional carbon fibers based on pitch and polyacrylonitrile (PAN) are also included. ( a ) Mechanical property. ( b ) Electrical property. Full size image The electrical conductivities of neat CNT fibres reported in the literature also show significant discrepancy, varying from <10 to <1000 S cm −1 , as summarized in Supplementary Table 1 and Fig. 6b . Aerogel [24] and solution-originated fibres [30] were reported to have high κ values of 8.3 × 10 3 S cm −1 . The highest κ value measured is 2.9 × 10 4 S cm −1 for the recently reported fibre spun from a solution [13] , which is slightly higher than that of ~2 × 10 4 S cm −1 for the present fibre containing impurities such as Fe particles and CNTs with a lower I G / I D . Common with these two high κ fibres is high packing density, which was achieved by extrusion and rolling, respectively. Highly packed CNTs have low contact resistance, therefore, leading to fibres of high conductivity. Nevertheless, it should be noted that the present fibre has mechanical properties much better than the solution-spun fibre ( σ b : 4.34 versus 1.0 GPa, δ : 10 versus 1.4%). As the present fibre-like ribbon has a thin thickness, it is meaningful to compare its properties with those for CNT films. The mechanical and electrical properties of CNT films made by different methods are listed in Supplementary Table 2 , and graphically illustrated in Supplementary Fig. 5 . As shown, the highest tensile strengths for previous CNT films are up to 2 GPa, which is coupled with very low conductivities, and the highest conductivities are up to 10 4 S cm −1 , but with a very low strength. These properties are apparently much inferior to the concurrent possession of high strength of 3.76–5.53 GPa and high conductivity of 1.82–2.27 × 10 4 S cm −1 shown by the present sample. The further highlight of the present CNT assembly is its high competitivity with CFs. First, its production method is simpler, commending it on both cost and environmental grounds, than the complicated and high energy-consuming methods used for production of CFs [1] . Second, the strength of the present CNT assembly (3.76–5.53 GPa) has reached the level of commercially available high-strength CFs. Even when 10 layers of CNT cylinders were stacked on each other and then rolled to have a thickness comparable to the diameter of CFs (~7 μm), preliminary results still showed a high ultimate strength of 4.0 GPa for the new assembly ( Supplementary Fig. 6 ). This is the first time for a CNT assembly to make such an achievement in tensile strength. The current high-strength CFs are polyacrylonitrile-based, having strengths in the range of 3.5–5.5 (typically, T300: 3.5 GPa, T700S: 4.9 GPa, from Toray Co., although less common grades, H800 and H1000, with higher strength are also available, but from heat treatment at extremely high temperature; Supplementary Table 1 ). But, such CFs have a ductility as low as 2% due to the difficult interplane slip. This ductility is much lower than that for CNT fibres (10%) in which intertube sliding and even innertube stretching are widely available. The high ductility, combined with high failure strength, means that the work needed to break the CNT fibres (called toughness) is also high, which will increase the safety factor of CNT fibre composite structures by preventing catastrophic failure. The high-strength CFs not only have a low ductility but a low electrical conductivity as well. Among various kinds of CFs, the pitch-based ones have the highest conductivity, being in the range of (0.1–1) × 10 4 S cm −1 , which is still lower than CNT fibres. Furthermore, such CFs had lower strengths (1–3 GPa) and almost no ductility (<1%). Thus, the present CNT assembly may compete with CFs for high-end uses, especially in weight-sensitive applications demanding combined electrical and mechanical functionalities. A few examples to note are light-weight, high-strength and multifunctional composites for military and aerospace structure components and electrical conductors for power transmission lines [7] . The tensile strength and electrical conductivity reported here are still one and two orders of magnitude lower than those theoretical values predicted for individual single-walled CNTs, respectively. To narrow the gap further, the structural parameters such as length, diameter and alignment of CNTs should be better controlled. For strength improvement, the intertube load transfer may be manipulated by already reported methods such as electron irradiation [31] , [32] , chemical treatment [33] and polymer impregnation [34] , [35] , [36] , forming primary bonds between CNTs, which are much stronger than Van der Waals interactions. For conductivity improvement, tube chirality should be particularly tailored [37] , and iodine doping [13] , [38] and metal coating [39] , [40] may be imposed. However, it should be noted that all these modifications may result in gain of one property but loss of another, and the theoretical properties may not be reachable because of the inevitable presence of defects within CNTs and between their surfaces. In summary, a cylindrical film consisting of thin-walled CNTs formed at the downstream of a tube reactor, and could be continuously blown into open air environment. The CNT cylinder could be condensed in water or alcohol and spun as a fibre over the time length as long as the reaction solution was supplied. In order to densify the fibre, pressurized rolling was applied, which led to improvements of mechanical and electrical properties by more than one order of magnitude. Mainly due to severe densification, the CNT assembly after rolling had an excellent combination of high strength (4.34 GPa), high ductility (10%) and high conductivity (2 × 10 4 S cm −1 ), which appears to be unrivalled by any other fibres and films currently available. The observed drastic improvements point to considerable potential of CNT materials processed by pressurized rolling in any CNT laboratory of the world, and the unrivalled combination makes CNT fibres competitive to CFs for high-end uses. Synthesis of hollow cylindrical CNT assembly The hollow cylinder-like CNT assembly was continuously synthesized at 1150–1300 ° C in a horizontal furnace using an alundum tube and nitrogen as the reactor and carrier gas, respectively. The precursor solution consisted of a liquid feedstock of carbon source (typically, ethanol) with dissolved ferrocene and thiophene. This solution was injected into the reactor at a rate of 2–10 ml min −1 , and carried into the high-temperature zone by N 2 at a flow rate of 16–32 l h −1 . The cylindrical film formed on the inner side wall of the reactor at the downstream, and was driven out from the reactor to air atmosphere by the enclosed N 2 and gaseous products from the pyrolysis of the reaction solution. The inner diameter of the reactor ranged from 30 to 100 mm. The experimental results are reported mainly from reactors with smaller diameters, unless otherwise noted. Formation of CNT fibres The CNT cylinder floating in air was introduced into water for shrinking. For comparison, ethanol was also used for shrinking, but only occasionally for safety and environmental reasons. The fibre formed in water was pulled out below a rotating stainless steel rod and winded onto a mandrel. The winding rate was properly adjusted to match the running rate of the cylinder but always slightly higher than the running rate to improve CNT alignment by continuous stretching. The winding rate was 2–20 m min −1 , depending on the specific experimental conditions. Mechanical rolling of CNT fibres In order to enhance the compactness of the winded fibre, we carried out pressurized rolling. Two rollers rotated synchronously, but at opposite directions. A load of several kilograms was applied on the top roller to ensure a highly pressurized contact with the bottom roller. The rotation of the rollers took in and drove out the fibre. The rolling was repeated for a number of times for microstructure and property optimization. In each run, the fibre-like ribbon was oriented so as to have it rolled at its thickness direction. Characterization and analysis CNTs were characterized by thermo-gravimetric analysis (Netzsch Model STA 409 PC, heating rate of 10 °C min −1 and a constant air flow of 20 ml min −1 ), high-resolution transmission electron microscopy (JEOL-2010F, accelerating voltage of 200 kV), field emission scanning electron microscopy (FEI Sirion 200) and Raman spectroscopy (Raman, Renishaw inVia, excitation wavelength of 514 nm). The width of CNT fibre-like ribbons was measured by SEM, S-3400N. The pore structure of CNT assemblies before rolling was examined by transmission electron microscopy (FEI Tecnai G2 Spirit BIOTWIN, accelerating voltage of 120 kV). In this case, a CNT fibre was embedded in epoxy resin first. After curing, the sample was cut perpendicular to the fibre axis. For thickness measurement by SEM, a CNT ribbon was vertically attached on the sample stage with conductive adhesive glued on two sides. The stage was carefully rotated until a clear cross section could be visualized. The degree of alignment of CNTs in the ribbon, y , was measured by wide-angle X-ray diffraction on a Rigaku D/Max-2550 PC X-ray diffractometer operated with a Cu K α radiation target at 40 kV and 350 mA (scanning range: 6–50°, interval: 0.02°, rate: 5°min −1 ). Both as-spun and rolled samples, consisting of approximately 50 segments cut directly from the spindles, were measured. The value of y was calculated from the equation: y =(1–Σ h i /360) × 100%, in which h i is the full width at the half maximum of i peak for (002) diffraction. Tensile and resistance tests The tensile tests were performed on a fibre tensile tester (XS(08)X-15, Shanghai Xusai Co., China), which is equipped with a deformation loading system and a force measuring system with a maximum force of 15 N and precision of 0.01 cN. The digital output of the load cell was routinely checked by hanging on different known weights, and the displacement of the cross head was inspected by optical means. The fibres used for tensile measurement were directly fixed on the tester with clamps at both ends after the tester was calibrated. After the upper part of the fibre had been clamped, a small weight (0.5 g) was applied on the lower end, to ensure that the sample was taut. Then, the lower part of the fibre was clamped at the position to have a designed GL. The tensile testing was usually performed at a displacement rate of 20 mm min −1 and a GL of 10 mm, which corresponds to an engineering strain rate of ~3.33 × 10 −2 s −1 . To examine the uniformity along its length, the fibre was also tested at other GLs (1, 5 or 20 mm). The electrical resistance of CNT fibres was measured by a four-point probes metre (SX1944, Suzhou Baishen Technology Co., China). The electrical conductivity κ was calculated through κ = L / RA , where L , R and A are the length, resistance and cross-sectional area of CNT fibres, respectively. For both tensile and resistance tests, the measurements were repeated many times, usually metres apart along the length of the fibre, to get an average value. How to cite this article : Wang, J. N. et al. High-strength carbon nanotube fibre-like ribbon with high ductility and high electrical conductivity. Nat. Commun. 5:3848 doi: 10.1038/ncomms4848 (2014).